Mineral phosphorus drives glacier algal blooms on the Greenland Ice Sheet Melting of the Greenland Ice Sheet is a leading cause of land-ice mass
                loss and cryosphere-attributed sea level rise. Blooms of pigmented glacier ice algae
                lower ice albedo and accelerate surface melting in the ice sheet’s southwest sector. Although glacier ice algae cause up to 13% of the surface melting in this region,
                the controls on bloom development remain poorly understood. Here we show a direct
                link between mineral phosphorus in surface ice and glacier ice algae biomass through
                the quantification of solid and fluid phase phosphorus reservoirs in surface
                habitats across the southwest ablation zone of the ice sheet. We demonstrate that
                nutrients from mineral dust likely drive glacier ice algal growth, and thereby
                identify mineral dust as a secondary control on ice sheet melting. The Greenland Ice Sheet (GrIS) comprises only 11.2% of land ice on
                        Earth [1] , yet surface melting and ice-calving from the
                GrIS accounted for 37% of cryosphere attributed sea level rise between 2012 and
                        2016 [2] . Mass loss is predominantly determined by the
                incoming shortwave radiation flux [3] , [4] modulated by surface albedo [5] . There has been a ~40% increase in surface
                melting and runoff from the GrIS over the last quarter of a
                        century [6] as a north−south oriented band of low-albedo ice,
                known as the Dark Zone, has developed along the western margin of the ice
                        sheet [7] . Albedo depends on the physical structure of
                surface ice [8] and the presence of light absorbing particulates (LAP), which include pigmented
                glacier snow and ice algae, black carbon (BC), and mineral
                        dust [7] . Glacier ice algae (hereafter glacier algae) produce
                photoprotective phenolic pigments [9] , [10] , [11] , [12] , [13] , [14] that lower ice sheet albedo on the
                landscape-scale, thereby contributing to melting [15] , [16] . Glacier algae were calculated to be
                directly responsible for 9−13% of the surface melting in the Dark Zone in
                        2016 [16] , and there are comparable indirect effects due
                to water retention and changes to ice crystal fabric as a result of algal
                        growth [8] . While glacier algal blooms can cover up to 78%
                of the ice surface [16] , they exhibit a high degree of interannual
                variability in intensity and spatial extent [7] that is yet to be understood. Thus, there is a pressing need to better quantify the parameters that control
                glacier algal growth and constrain the impact of these blooms on ice sheet albedo,
                melting, and contributions to sea-level rise. Here we demonstrate, through nutrient
                addition experiments and spatially resolved mineralogical and geochemical data, that
                phosphorus is a limiting nutrient for glacier algae in the Dark Zone. We identify
                phosphorus-bearing minerals (hydroxylapatite) as the likely phosphorous nutrient
                source fueling glacier algal blooms. We also disentangle the biogeochemical controls
                on ice sheet darkening by characterizing the source, composition, and nutrient
                delivery capacity of mineral dust. These results, in combination with nutrient
                addition experiments, demonstrate that phosphorus from mineral dust is a limiting
                nutrient for algal blooms in the Dark Zone. Phosphorus is a limiting nutrient for glacier algae Glacier algal blooms were studied at five sites along a transect
                    across the ablation zone in southwest GrIS (Fig. 1a ). Surface snow and ice samples were collected at locations
                    ~33−130 km from the ice margin in 2016 and 2017 (Sites 1−5), with reference
                    rocks collected near the Russell Glacier terminus in 2018 (Site 6;
                        Fig. 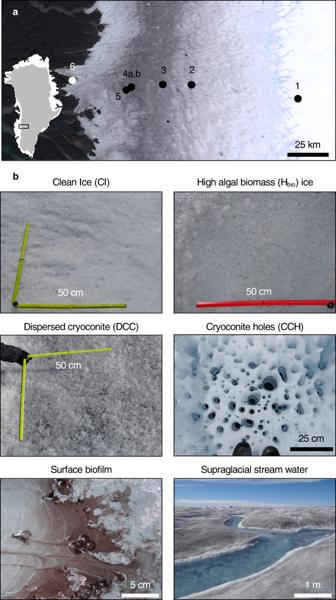Fig. 1: Sample collection locations and habitats on the Greenland
                                    Ice Sheet. aSample collection
                                    sites 1–5 across the ablation zone in southwest Greenland Ice
                                    Sheet and rock sample collection site 6 near the terminus of
                                    Russell Glacier viewed using Sentinel-2 imagery (cloud-free
                                    composite of all acquisitions between 01/07/2016 and
                                    31/08/2016);bphotographs of
                                    surface ice habitats: clean ice (CI), high algal biomass ice
                                        (Hbio), dispersed cryoconite ice
                                    (DCC), cryoconite holes (CCH), surface biofilm, and supraglacial
                                    stream water. 1a , Supplementary
                        Table 1 ). Targeted surface
                    habitats included clean ice (CI; free of macroscopically visible LAP), high
                    algal biomass (H bio ) ice, H bio snow, dispersed cryoconite (DCC) ice, cryoconite holes (CCH), a floating
                    biofilm, and supraglacial stream water (Fig. 1b ). To identify potential nutrient limitations on glacier
                    algal growth, we carried out a series of soluble nutrient addition incubation
                    experiments at Site 4b using H bio ice
                        (8.0 ± 2.1 × 10 3 cells mL −1 ) that was melted in the dark over
                    24 h, and re-incubated for 120 h across five treatments (phosphate, nitrate,
                    ammonium, phosphate+nitrate+ammonium (+ALL), control). Concomitantly, the health
                    and productivity of glacier algae assemblages were monitored using rapid light
                    response curves [17] performed with pulse amplitude modulation
                    (PAM) fluorometery at 24, 72, 120 h. A significant response to phosphorus
                    addition was apparent after 120 h of incubation (Fig. 2a ), achieving the maximum quantum efficiency ( F v / F m : inverse proxy of microalgae stress)
                    and maximum rates of electron transport ( rETR max : proxy for photosynthesis rate). Both parameters displayed positive responses to increased P availability
                        (PO 4 3- and +ALL
                    treatments) compared to other treatments (Fig. 2b,
                        c ). Specifically, after 120 h there were no significant
                    differences between the rETR max measurements made for the
                    phosphate and +ALL treatments, and both of these treatments were significantly
                    higher than each of the control, ammonium, and nitrate treatments, with no
                    significant differences between the latter three treatments (Supplementary
                        Tables 2 and 3 ). These results indicate that phosphorus was
                    the limiting nutrient for glacier algal growth at Site 4b. No significant
                    differences in photophysiological parameters were apparent after 24 or 72 h
                    across treatments (Supplementary Tables 2 and 3 ,
                    Supplementary Fig. 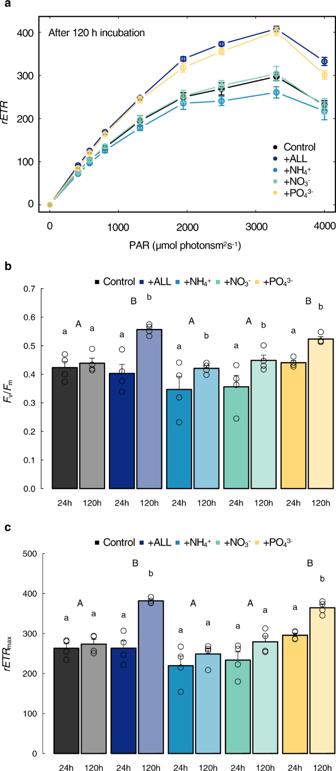Fig. 2: Glacier algal photophysiological response to nutrient
                                    addition. aRelative electron
                                    transport rates (rETR)
                                    measured during rapid light curves (RLCs) following 120 h
                                    incubation,bmaximum quantum
                                    efficiency in the dark-adapted state (Fv/Fm) andcmaximum electron
                                    transport rate (rETRmax) after 24 and
                                    120 h incubation. All plots show mean ±SE,n= 4.b,clower and
                                    upper case letters denote homogeneous subsets identified from
                                    two-way ANOVA analysis of respective parameters in relation to
                                    duration and nutrient treatment, respectively. Two-way ANOVA
                                    results comparing treatments:F4,30= 6.48,P= 0.000699, and time points (24
                                    vs 120 h):F4,30= 28.75,P= 0.00000839 forFv/Fm. Two-way
                                    ANOVA results comparing treatments:F4,30= 16.71,P= 0.000000264, and time points:F4,30= 35.07,P= 0.00000174 forrETRmax. The
                                    results of Tukey HSD tests comparingFv/FmandrETRmaxresults for
                                    treatments at 24 and 120 h can be found in Supplementary
                                        Tables2and3. 1 , data for 72 h
                    not shown). The delayed response to phosphorus addition until 120 h suggests a
                    mechanism of phosphate storage sufficient to sustain glacier algal productivity
                    for ~5 days, which is similar in duration to the doubling time of 5.5 ± 1.7 days
                    reported for glacier algal populations from this region [15] . 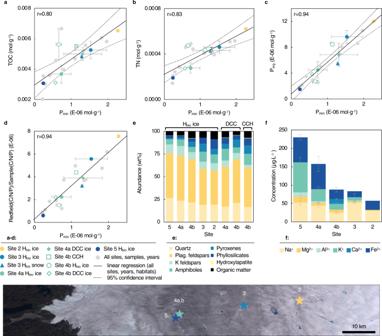Fig. 3: Dark Zone particulate matter nutrient concentrations,
                                    mineralogy, and major cation concentrations in associated
                                    meltwater. Pminconcentration in
                                    particulates plotted againstatotal organic carbon (TOC),btotal nitrogen (TN),corganic
                                    phosphorus (Porg), anddmolar
                                        C:N:Porgratio normalized to the
                                    Redfield ratio (C:N:P 106:16:1). Linear regression and r-values
                                    (Pearson’s product-moment correlation) correspond to all data
                                    points from all sites (gray dots).eRelative mineral and organic matter abundances
                                    across the ablation zone, including hydroxylapatite (bright
                                    yellow);fmajor cation
                                    concentrations in meltwater from Hbioice
                                    across the ablation zone. Hbioice: high
                                    algal biomass ice; DCC ice: dispersed cryoconite ice; CCH:
                                    cryoconite hole. Ina–d: colored points: mean values for
                                    different sites, habitats, and years, ±SE (2016: solid fill;
                                    2017: white-fill); solid line: linear regression; thin dashed
                                    lines: 95% confidence interval. Site 2
                                        Hbioicen= 1; Site 3 Hbioicen= 2; Site 3
                                        Hbiosnown= 1; Site 4a Hbioicen= 5; Site 4a DCC icen= 2; Site 4b
                                        Hbioicen= 2; Site 4b DCC icen= 1; Site 4b CCHn= 1; Site 5 Hbioicen= 1. Ine: Hbioice:
                                    site 5:n= 1; site 4an= 5; site 4b:n= 4; site 3:n= 2; site 2n= 1; DCC ice: site 4an= 4; site 4bn= 1; CCH site 4bn= 1. Inf: site 5n= 6; site 4an= 5; site 4bn= 3; site 3n= 2; site 2n= 1. 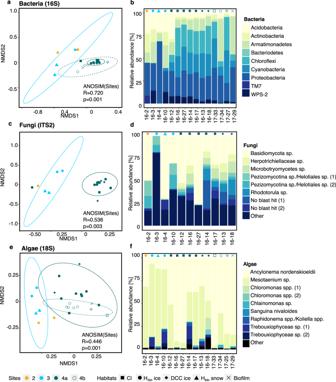Fig. 4: Composition of bacterial, fungal, and algal communities in
                                    surface habitats across the Dark Zone. NMDS plots showing the sample similarities for bacteria
                                        (a), fungi (c), and algae (e) and their respective community compositions
                                    based on relative abundances (b,d,f). Sites are represented by colors
                                    and habitats by point shapes. Samples cluster according to sites
                                    and dashed lines represent the 95% confidence interval. All
                                    samples with a sufficiently high number of sequences were used
                                    for the NMDS plots, whereas representative samples across sites
                                    and habitats were selected for the bar charts (details in
                                    Supplementary Tables9–13). Due to the slow
                    doubling time of glacier algae, it is not surprising that a significant increase
                    in cell counts was not measured over the 120 h experiment (Supplementary
                        Table 4 ). Luxury uptake of
                    phosphorus is common among microorganisms, with phosphorus stored
                    intracellularly as polyphosphates that can act as an extraneous source under
                    limiting conditions [18] . Such a storage mechanism would be
                    beneficial for glacier algae inhabiting the oligotrophic surface ice
                    environments of the GrIS Dark Zone. The lack of a photophysiological response to
                    the addition of nitrate or ammonium suggests that glacier algae are not limited
                    by N. Although our measurements of dissolved inorganic N in surface ice and snow
                    samples were low or below detection limit (Supplementary Table 8 ), inorganic and organic N have been
                    documented in H bio ice habitats in concentrations of 1.0
                    and 14 µM, respectively [19] , indicating that N is available in the
                        system. Fig. 1: Sample collection locations and habitats on the Greenland
                                    Ice Sheet. a Sample collection
                                    sites 1–5 across the ablation zone in southwest Greenland Ice
                                    Sheet and rock sample collection site 6 near the terminus of
                                    Russell Glacier viewed using Sentinel-2 imagery (cloud-free
                                    composite of all acquisitions between 01/07/2016 and
                                    31/08/2016); b photographs of
                                    surface ice habitats: clean ice (CI), high algal biomass ice
                                        (H bio ), dispersed cryoconite ice
                                    (DCC), cryoconite holes (CCH), surface biofilm, and supraglacial
                                    stream water. Full size image Fig. 2: Glacier algal photophysiological response to nutrient
                                    addition. a Relative electron
                                    transport rates ( rETR )
                                    measured during rapid light curves (RLCs) following 120 h
                                    incubation, b maximum quantum
                                    efficiency in the dark-adapted state ( F v / F m ) and c maximum electron
                                    transport rate ( rETR max ) after 24 and
                                    120 h incubation. All plots show mean ±SE, n = 4. b , c lower and
                                    upper case letters denote homogeneous subsets identified from
                                    two-way ANOVA analysis of respective parameters in relation to
                                    duration and nutrient treatment, respectively. Two-way ANOVA
                                    results comparing treatments: F 4,30 = 6.48, P = 0.000699, and time points (24
                                    vs 120 h): F 4,30 = 28.75, P = 0.00000839 for F v / F m . Two-way
                                    ANOVA results comparing treatments: F 4,30 = 16.71, P = 0.000000264, and time points: F 4,30 = 35.07, P = 0.00000174 for rETR max . The
                                    results of Tukey HSD tests comparing F v / F m and rETR max results for
                                    treatments at 24 and 120 h can be found in Supplementary
                                        Tables 2 and 3 . Full size image Phosphorus limitation decreases with increasing mineral
                    phosphorus To assess potential phosphorus sources, sequential P extractions
                    were conducted (Steps I, III, IV, and V from Ruttenberg, et
                            al. 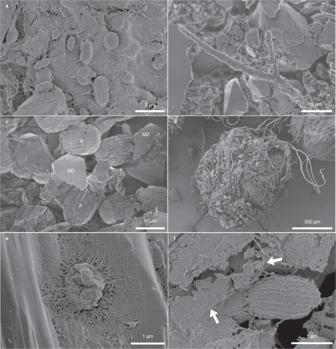Fig. 5: Scanning electron micrographs of cell-mineral associations
                                    in Dark Zone surface habitats. Scanning electron microscopy (SEM) micrographs showingabacteria,bfungi, andcglacier algae that comprise the Dark Zone
                                    microbial community. Microbes inc) Hbioice are more
                                    disseminated than those indcryoconite granules. In all surface ice habitats, exopolymer
                                    enables microbial cells toeadhere to mineral surfaces, andftrap and bind mineral grains (arrows). IncA: algal cells, MD:
                                    mineral dust. Images ina–fare
                                    representative of then= 12
                                    samples observed using SEM. [20] ) and revealed that organic phosphorus
                        (P org ) accounted for up to 86% of the solid-phase P
                    in H bio ice (Supplementary Table 5 ), with exchangeable
                        (P exch ; <31%) and mineral phosphorus
                        (P min ; 17%) comprised the remaining solid-phase P.
                    Molar concentrations of total organic carbon (TOC), total nitrogen (TN), and
                        P org all showed a positive correlation with
                    particulate P min concentrations (Fig. 3a–c , Supplementary Note 1 , Supplementary Table 5 ). The solid-phase nutrient ratios
                        (C:P org , C:N, and N:P org ),
                    which reflect the nutrient pools in the algal dominated biomass, indicate P as
                    the limiting nutrient, particularly when compared to Redfield ratios (C:N:P
                    106:16:1; Supplementary Fig. 2 ) [21] . Normalizing solid-phase C:N:P molar
                    ratios to Redfield C:N:P clearly shows that samples containing higher
                    concentrations of P min were closer to achieving Redfield
                    ratio concentrations of organic nutrients, thereby providing an indication of
                    potential nutrient limitation (Fig. 3d ). The ratio of TOC:N:P org measured in site 4
                        H bio particulates ranged between 690:48:1
                    and 2615:196:1, which mirrors the dissolved organic nutrient ratios reported in
                    Holland, et al. [19] (DOC:DON:DOP = 2017:117:1). In the present
                    study, we find that as the concentration of solid-phase
                        P min increases, the C:N:P ratio decreases and
                    approaches the ideal Redfield C:N:P ratio. This trend was observed for
                    solid-phase samples from all habitats and locations sampled in both
                        years. Fig. 3: Dark Zone particulate matter nutrient concentrations,
                                    mineralogy, and major cation concentrations in associated
                                    meltwater. P min concentration in
                                    particulates plotted against a total organic carbon (TOC), b total nitrogen (TN), c organic
                                    phosphorus (P org ), and d molar
                                        C:N:P org ratio normalized to the
                                    Redfield ratio (C:N:P 106:16:1). Linear regression and r-values
                                    (Pearson’s product-moment correlation) correspond to all data
                                    points from all sites (gray dots). e Relative mineral and organic matter abundances
                                    across the ablation zone, including hydroxylapatite (bright
                                    yellow); f major cation
                                    concentrations in meltwater from H bio ice
                                    across the ablation zone. H bio ice: high
                                    algal biomass ice; DCC ice: dispersed cryoconite ice; CCH:
                                    cryoconite hole. In a – d : colored points: mean values for
                                    different sites, habitats, and years, ±SE (2016: solid fill;
                                    2017: white-fill); solid line: linear regression; thin dashed
                                    lines: 95% confidence interval. Site 2
                                        H bio ice n = 1; Site 3 H bio ice n = 2; Site 3
                                        H bio snow n = 1; Site 4a H bio ice n = 5; Site 4a DCC ice n = 2; Site 4b
                                        H bio ice n = 2; Site 4b DCC ice n = 1; Site 4b CCH n = 1; Site 5 H bio ice n = 1. In e : H bio ice:
                                    site 5: n = 1; site 4a n = 5; site 4b: n = 4; site 3: n = 2; site 2 n = 1; DCC ice: site 4a n = 4; site 4b n = 1; CCH site 4b n = 1. In f : site 5 n = 6; site 4a n = 5; site 4b n = 3; site 3 n = 2; site 2 n = 1. Full size image Using our particulate mass loading data, glacier algae cell
                            dimensions [14] , the algal cell-nutrient content calculation
                    in Montagnes, et al. [22] , and accounting for the abundance of
                    heterotrophic bacteria the Dark Zone [23] , we have calculated that the TOC and TN
                    measured in our H bio ice samples translate to glacier
                    algal cell concentrations of 1.2–5.6 × 10 4 cells mL −1 (see Supplementary Note 2 for calculation details). These values are
                    comparable to glacier algal cell abundances reported in the
                            area [11] , [15] , [24] and consistent with the average glacier
                    algal cell abundance of 2.9 ± 2.0 × 10 4 cell mL −1 we reported in Cook, et
                            al. [16] for the same region in 2016. Note, our
                    calculated cell counts may be a slight overestimation due to some of the
                    measured TOC being present in the form of microbial exopolymer or dead cells. This calculation does, however, reveal that <1% of the total TOC is
                    present in the form of bacteria, thereby confirming that the majority of the
                    solid-phase nutrients measured on the ice surface are found in glacier
                    algae. 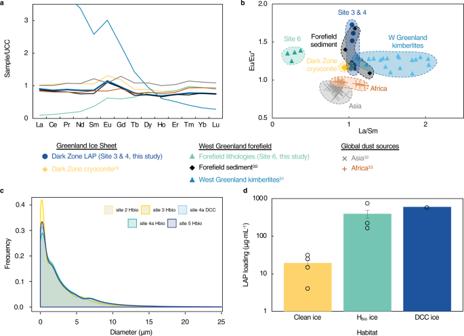Fig. 6: Rare Earth element signature and grain size distribution
                                    for mineral dust in Dark Zone particulates. a,bRare Earth element (REE) normalized
                                    to the upper continental crust (UCC) compared to potential
                                    sources;cmineral dust size
                                    distribution; anddparticulate
                                    mass loading by habitat. Indplot shows mean ± SE, clean ice:n= 4 samples, high algal biomass ice
                                        (Hbio) ice:n= 3 samples, dispersed cryoconite (DCC) ice:n= 1
                                    sample. The measured P min is likely sourced from
                    trace hydroxylapatite
                        [Ca 5 (PO 4 ) 3 (OH); < 1.1 wt%],
                    which we have identified in Dark Zone surface ice dust using Rietveld
                            refinement [25] of powder X-ray diffraction (XRD) data
                    (Supplementary Table 6 ). The
                    mineralogy of the dust was dominated by plagioclase feldspars (41−54 wt%) and
                    quartz (18−30 wt%) (Fig. 3e ,
                    Supplementary Note 3 , Supplementary
                        Fig. 3 , Supplementary
                        Tables 6 and 7 ). Ferromagnesian phases including amphiboles
                    (4−14 wt%) and pyroxenes (<10 wt%), along with potassium feldspars
                    (3−12 wt%), micas (1−6 wt%), and kaolinite (<3 wt%) comprise the
                    remaining fraction. Nutrient biomining by supraglacial microbes The hydroxylapatite presents an important link between mineral dust
                    and glacier algal blooms because it contains bio-essential
                            phosphorus [26] . Mineral abundances and meltwater chemistry
                    together suggest increased mineral weathering with proximity to the ice sheet
                    margin; H bio ice closer to the margin (Sites 4 and 5)
                    contained lower abundances of ferromagnesian phases than inland sites, with the
                    corresponding meltwater enriched in dissolved major cations
                        (Na + , Mg 2+ ,
                        Al 3+ , K + ,
                        Ca 2+ , Fe 2+ )
                        (Fig. 3f , Supplementary
                        Note 4 , Supplementary
                        Table 8 ). Elevated concentrations
                    of soluble cations in H bio ice may be due to increased
                    rates of abiotic or biotic (heterotrophic bacteria or fungi) mineral dust
                    weathering, or through retention of cations via adsorption to negatively charged
                    cell exteriors. Examining the composition of the microbial communities along the
                    transect revealed that the algal (18 S), bacterial (16 S), and fungal (ITS2)
                    community compositions clustered according to sampling sites but exhibited
                    spatial variability across the Dark Zone (Fig. 4 , Supplementary Tables 9 – 13 ). All
                    communities showed a higher similarity within one site than within one habitat
                    (Supplementary Note 5 ), indicating an
                    association between the local geochemistry and microbiology. This is valid
                    across sampling years; 2016 and 2017 samples collected from Site 4 were more
                    similar than samples collected over three weeks in 2016 from Sites 2, 3, and 4a
                        (Fig. 4 ). Since Ancylonema nordenskioeldii and Mesotaenium sp. comprised between 66 and 99% of the
                    algal community in all samples (Supplementary Table 13 ), the assemblage of glacier algae used in the nutrient
                    addition experiments at site 4 was reasonably representative of the region. Collectively, the microbial community (Fig. 5a–c ) was intermixed with mineral dust and occurred as
                    disseminated particulates in H bio ice (Fig. 5c ) and aggregated cryoconite granules in DCC ice
                    and cryoconite hole material (Fig. 5d ). Microbial exopolymer enables cells to both adhere to mineral dust
                        (Fig. 5e ) and trap and bind mineral
                    grains (Fig. 5f ). Fig. 4: Composition of bacterial, fungal, and algal communities in
                                    surface habitats across the Dark Zone. NMDS plots showing the sample similarities for bacteria
                                        ( a ), fungi ( c ), and algae ( e ) and their respective community compositions
                                    based on relative abundances ( b , d , f ). Sites are represented by colors
                                    and habitats by point shapes. Samples cluster according to sites
                                    and dashed lines represent the 95% confidence interval. All
                                    samples with a sufficiently high number of sequences were used
                                    for the NMDS plots, whereas representative samples across sites
                                    and habitats were selected for the bar charts (details in
                                    Supplementary Tables 9 – 13 ). Full size image Fig. 5: Scanning electron micrographs of cell-mineral associations
                                    in Dark Zone surface habitats. Scanning electron microscopy (SEM) micrographs showing a bacteria, b fungi, and c glacier algae that comprise the Dark Zone
                                    microbial community. Microbes in c ) H bio ice are more
                                    disseminated than those in d cryoconite granules. In all surface ice habitats, exopolymer
                                    enables microbial cells to e adhere to mineral surfaces, and f trap and bind mineral grains (arrows). In c A: algal cells, MD:
                                    mineral dust. Images in a – f are
                                    representative of the n = 12
                                    samples observed using SEM. Full size image Heterotrophic bacteria [26] and fungi [27] can accelerate apatite
                    weathering beyond abiotic rates, thereby transferring solid-phase P to the
                    organic reservoir. This accounts for the lower P min concentration at sites hosting more prolific algal blooms (4 and 5), where a
                    higher proportion of P min has been transformed into
                        P org through bioweathering and algal biomass
                    accumulation. Glacier algal productivity outstrips that of associated
                    heterotrophic assemblages [23] , and likely drives recycling of
                    solubilized P. Site 4a H bio and DCC ice contained three
                    to four times more dissolved P than clean ice or supraglacial stream water
                    (Supplementary Table 8 ),
                    substantiating claims that P is retained in surface ice
                            habitats [19] . Microbes may similarly be utilizing mineral iron; ferromagnesian
                    minerals are less abundant in H bio ice than other
                    habitats, and decrease in abundance among H bio samples by
                    up to 60 % at sites hosting more prolific algal blooms (Fig. 3e ). Dissolved iron concentrations in
                        H bio ice show a concomitant inverse trend
                        (Fig. 3f , Supplementary
                        Table 8 ). Specifically, at Site
                    4a, the concentration of iron was two and four-time higher in
                        H bio ice (69 ± 20 μg L −1 )
                    than DCC ice (36 ± 5 μg L −1 ) and clean ice
                        (16 ± 13 μg L −1 ), respectively (Supplementary
                        Table 8 ). If iron is extracted as
                    a micronutrient, this has downstream implications for export of bioavailable
                    iron from the ice sheet to the marine system [28] . Mineral dust source and transport Our findings indicate that mineral dust facilitates glacier algal
                    bloom development by supplying the needed P to the supraglacial algal
                    communities. The REE (rare earth element) signatures of the mineral fraction in
                    our surface samples were used to assess dust source. The REE signatures were
                    homogenous and exhibited a positive Eu/Eu* anomaly analogous to local sources
                    (Supplementary Note 6 , Supplementary
                        Table 14 ) [29] , [30] , [31] thereby excluding distal sources
                    characterized by a negative Eu/Eu* anomaly (Asian [32] and
                            African [33] dust) as significant contributors
                        (Fig. 6a, b ). A local mineral source
                    means that the hydroxylapatite in our particulates was derived from
                    local apatite-bearing lithologies [34] . Local delivery of mineral dust to the
                    GrIS is consistent with ice core records that indicate delivery of Greenlandic
                    dust to the ice sheet during interglacial periods [35] . Furthermore, analysis
                    of the grain-size distribution of our particulate dust fractions revealed that
                    99% of all grains were <20 μm in diameter (Fig. 6c ), consistent with atmospheric transport
                    processes that are typically limited to mobilizing grains <20
                            μm [36] . Fig. 6: Rare Earth element signature and grain size distribution
                                    for mineral dust in Dark Zone particulates. a , b Rare Earth element (REE) normalized
                                    to the upper continental crust (UCC) compared to potential
                                    sources; c mineral dust size
                                    distribution; and d particulate
                                    mass loading by habitat. In d plot shows mean ± SE, clean ice: n = 4 samples, high algal biomass ice
                                        (H bio ) ice: n = 3 samples, dispersed cryoconite (DCC) ice: n = 1
                                    sample. Full size image Mineral dust is a second-order control on Dark Zone ice albedo We documented that H bio ice contained
                    >30× more particulate mass per volume of ice than clean ice
                        (394 ± 194 μg mL −1 vs
                        19 ± 6 μg mL -1 ; Fig. 6d ). Mineral dust accounted for 94.2 ± 0.5 wt% of these
                    particulates (dry mass) in H bio and DCC ice, with the
                    organic matter comprising the remaining fraction (Fig. 3e , Supplementary Table 5 ). In spite of its dominance by mass, mineral dust is not
                    the primary cause of ice surface darkening in the GrIS Dark Zone. In situ
                    spectral reflectance measurements at Site 4 combined with refractive index and
                    mineral dust grain-size distribution measurements in a radiative transfer model
                    indicate that mineral dust has a negligible effect on albedo reduction compared
                    to pigmented glacier algae [16] . Rather, our findings indicate that the
                    presence of P min may have a second-order effect on
                    albedo. If this is the case, it follows that the spatial extent and melt rate of
                    P-bearing ice may in part constrain the spatial distribution of the algal blooms
                    producing the darkening observed on the landscape-scale. The limited first order effect of minerals on albedo is likely due
                    to dark-colored ferromagnesian phases (7−21 wt%) being intermixed with felsic
                    phases (79−93 wt%), namely feldspars and quartz, which are adept at scattering
                    light. The measured refractive index of the dust [16] indicates that light
                    scattering by felsic mineral grains supersedes light absorption by their
                    ferromagnesian counterparts. Note, these findings may not apply to all
                    locations; mineral dust can lower snow and ice albedo in
                            glacier [37] and ice sheet
                            environments [38] , [39] . This is dependent on the bulk complex
                    refractive index of the dust, which is a product of dust composition and
                    grainsize. This is compounded by factors such as the distribution of dust within
                    the ice matrix, mass mixing ratio, ice grain size and shape, and ambient
                    illumination conditions [40] . The high proportion of felsic mineral
                    grains may also indirectly contribute to albedo reduction via lensing of
                    pigmented algal cells in the same manner that mineral grains enhance light
                    absorption by black carbon nanoparticles through
                            lensing [41] . This effect depends on the structure and
                    mixing ratio of heterogeneous LAP aggregates in snow and ice. Its potential to
                    contribute to ice sheet albedo reduction remains unexplored. Microbes, minerals, and melting: a positive feedback system Previous studies have made links between snow algae and mineral
                    derived nutrients [42] , [43] , [44] , demonstrated that snow
                    algae respond to the addition of fertilizer [45] , and inferred that
                    glacier algal abundance correlate with mineral dust
                            loading [24] . Here we demonstrate how glacier algae
                    respond in situ to the addition of specific nutrients and link this response to
                    collocated nutrient-bearing mineral dust. Our findings demonstrate that mineral
                    nutrient availability is a second-order control on albedo by modulating glacier
                    algal bloom development. Comparable datasets spanning the GrIS are therefore
                    required to incorporate mineral dust as a factor in the positive feedback
                    between algal growth and surface melting. Algae induced melting liberates
                    ice-bound dust, from which heterotrophs can extract micronutrients. Recycled
                    nutrients augment glacier algal blooms, thereby further reducing albedo and
                    promoting additional melting. Furthermore, trapping and binding of mineral dust
                    by microbial exopolymers (Fig. 5f ),
                    helps retain valuable nutrients in the ice habitat. Notably, the glacier algal
                    biofilm contained the highest abundance of hydroxylapatite of all samples
                    (1.1 wt%; Supplementary Table 6 ),
                    suggesting preferential entrapment of hydroxylapatite in these complex microbial
                    colonies. Microbial retention of mineral dust reinforces the biological-albedo
                    reducing feedback by prolonging colocation of algae and essential nutrients on
                    the ice surface. Nevertheless, factors controlling the timing, spatial extent, and
                    intensity of algal blooms remain knowledge gaps limiting our ability to project
                    biological albedo reduction and melt. Bloom initiation depends on bare ice
                    exposure following snowpack retreat, as indicated by glacier algal cell counts
                    for the same locations [9] , and the fact that growth of cryophilic algae
                    can be stimulated by the presence of liquid water [45] . It is essential to
                    constrain the timing of bloom development following snowpack retreat because
                    satellite imagery indicates that surface darkening occurs within days of snow
                            clearance [7] . Since 2000, the melt season in the GrIS Dark
                    Zone has progressively started earlier, lasted longer, and exhibited greater
                    albedo reduction [7] , [46] . Years experiencing earlier winter snowpack
                    retreat yield more expansive algal blooms [47] . The higher
                        P min measured at inland sites (2 and 3) indicate that
                    these locations are geochemically primed to host future glacier algal blooms. These trends may be exacerbated by increased atmospheric delivery of mineral
                    dust to the ice sheet through increased windblown dust from exposed forefield
                            lithologies [48] , and by projected increased snowfall over
                    the GrIS [49] . The complexity of this rapidly changing Arctic system makes it
                    difficult to anticipate future changes to ice sheet albedo, melt rates, and
                    contributions to sea level. Our data provide a quantitative link between
                    mineral-derived nutrients and glacier algae blooms, and demonstrate that mineral
                    dust is an essential nutrient source for glacier algae. This biogeochemical
                    process must therefore be incorporated into predictive models thereby improving
                    our understanding of how glacier algal blooms will contribute to ice sheet
                    melting in the future. Sample collection and processing Surface snow and ice samples were collected along a transect across
                    the ablation zone of the southwestern margin of the Greenland Ice Sheet during
                    the 2016 (July 27–August 17) and 2017 (June 1–28) melt seasons
                        (Fig. 1 ). Site 4 was the basecamp
                    location in both seasons, differentiated as 4a (2016) and 4b (2017). Sites 1, 2,
                    3, and 5 were sampled only in 2016. The data presented are for samples
                    representing a range of surface snow and ice habitats. The clean snow sample
                    (GR16_1) collected at site 1 provides a reference for snow chemistry from the
                    accumulation zone. The sample did not contain sufficient particulate mass for
                    solid-phase chemical and mineralogical analyses. The collected samples were
                    classed into the following categories based on macroscopically visible
                    characteristics: clean snow ( n = 1), clean
                    surface ice (CI, n = 4), high algal biomass
                    ice (H bio ; n = 19),
                    high algal biomass snow ( n = 2), and
                    dispersed cryoconite ice (DCC; n = 5). In
                    addition, supraglacial stream water ( n = 2),
                    a sample of cryoconite hole (CCH) material ( n = 1), a cryoconite hole layer from an ice core ( n = 1), and a floating algal biofilm ( n = 1) were collected. Details of sample types and
                    collection locations are in Supplementary Table 1 . Clean was defined as surface snow and ice containing no
                    macroscopically visible particulates, H bio ice and snow
                    consisted of surface ice and snow containing visible glacier algal and
                    particulate material, and DCC consisted of ice surfaces covered in disseminated
                    particulate material from melted out cryoconite holes. Cryoconite hole material
                    was sampled to provide a biogeochemical reference for the DCC samples. The
                    biofilm sample consisted of a semi-coherent slick of aggregated microbial and
                    particulate material floating on the surface of ponded meltwater. Ice and snow
                    samples were collected from the top 3–5 cm of surface into sterile plastic bags,
                    melted at ambient temperatures (5–10 °C) (details in [50] , [51] ). Aliquots of filtered melted samples
                    were processed as described below for fluid chemistry analyses. While on the
                    ice, melted samples were filtered through glass fiber filters (GFF, pore size:
                    0.7 μm), from which the accumulated LAP were removed using a stainless steel
                    spatula. The collected solid LAP were air-dried and stored in glass
                    vials. Three rock samples representing lithologies in the catchment area
                    draining the west Greenland Ice Sheet were collected from outcrops near the
                    terminus of Russell Glacier (site 6 in Fig. 1a ). These samples provided a local rare Earth element
                    signature for comparison to that of the particulate samples, as described
                    below. Nutrient addition experiments A nutrient addition incubation experiment was performed during the
                    2017 ablation season at our base camp location (Site 4) to determine the
                    limiting nutrients for glacier algal assemblages. Five, 20 × 20 × 2 cm depth
                    surface ice areas containing a conspicuous loading of glacier algae were sampled
                    on June 22 nd 2017 into sterile Whirl-Pak bags, and
                    melted in the dark for 24 h under ambient on-ice conditions (5–10 °C). These
                    samples were used as the inoculum for the incubation experiments and had algal
                    counts of 8.0 ± 2.1 × 10 3 cells mL −1 (mean ± SD, n = 5). Algal cells were counted using a modified
                    Fuchs-Rosenthal haemocytometer (Lancing, UK) on a Leica DM 2000 epifluorescence
                    microscope with attached MC120 HD microscope camera (Leica, Germany). The
                    inoculum was incubated in 30 mL microalgal culturing flasks (Corning, UK) in
                    quadruplicates across five nutrient treatments: control (no nutrient addition),
                        +NH 4 + (10 µM final
                    concentration), +NO 3 − (10 µM
                    final concentration), +PO 4 3− (10 µM final concentration), and +ALL nutrients (10 µM of each
                        NH 4 and NO 3 ; 2 µM of
                        PO 4 to maintain a 10:1 N:P ratio across treatments). Nutrient concentrations were designed to provide ~10-fold ambient dissolved
                    inorganic nitrogen (DIN) and dissolved inorganic phosphorus (DIP) concentrations
                    previously reported for GrIS supraglacial ice [52] , [53] . After 24 h, 72 h, and 120 h, measurements of variable chlorophyll
                    fluorescence were performed on 3 mL incubation sub-samples with a WaterPAM
                    fluorometer and attached red-light emitter/detector cuvette system (Walz GmBH,
                    Germany). During the experiment, the ambient air temperature ranged between −4
                    and +4 °C. Rapid light response curves (RLCs) were performed to constrain
                    glacier algae photophysiology [17] , providing information on energy use
                    from limiting through to saturating levels of
                            irradiance [54] . All samples were dark-adapted for
                    20 minutes prior to RLC assessment, which was undertaken with a saturating pulse
                    of ca. 8,600 μmol photons m −2 s −1 for 600 ms duration and nine 20 s incremental
                    light steps ranging from 0 to
                        4000 μmol photons m −2 s −1 . Maximum quantum efficiency ( F v /F m ) was calculated from minimum
                        ( F o ) and maximum
                        ( F m ) fluorescence
                    yields in the dark-adapted state as F v /F m = ( F m − F o )/ F m . Electron transport through
                    photosystem II (PSII) was calculated from PSII quantum efficiency ( Y PSII ) in relative units
                        ( rETR = Y PSII × PAR × 0.5) assuming an equal division of photosynthetically
                    active radiation (PAR) between photosystem I and PSII. Analysis of rapid light
                    curves ( rETR ~ PAR)
                            followed [17] with iterative curve fitting in R (v.3.6.0)
                    and calculation of the relative maximum electron transport rate ( rETR max ), theoretical
                    maximum light utilization coefficient ( α ),
                    and light saturation coefficient ( E k ) following Eilers and
                            Peeters [55] . Statistical differences in
                    photophysiological parameters were assessed using two-way ANOVA with the fixed
                    variables of treatment (5 levels) and date (2 levels: 24 and 120 h) and the
                    interaction term, following tests of homogeneity of variance and normality of
                    distribution. Tukey HSD tests were used to assess statistically significant
                    differences in quantum efficiency and relative maximum electron transport rate
                    between nutrient treatments. Simultaneous to photophysiological measurements, a
                    further 5 mL of homogenized sample was fixed using 25% glutaraldehyde at 2%
                    final concentration and transported back to the University of Bristol, UK, to
                    assess glacier algal cell abundance (cells
                            ml −1 ) [9] , completed within 1 month
                    of sample return. Detailed statistical outputs and final cell count data can be
                    found in Supplementary Tables 2 – 4 ). Phosphorus extractions The phosphorus content of the H bio ice, DCC
                    ice, H bio snow, and CCH samples was determined using a
                    modified version of the SEDEX sequential extraction
                            protocol [20] . Steps I, III, IV, and V were completed as a
                    means of quantifying loosely bound/exchangeable P
                    (P exch ), mineral P (P min ), and
                    organic P (P org ). The extracted P was measured in the
                    fluid phase as described below for the melted ice samples. Detailed results can
                    be found in Supplementary Table 5 . Meltwater fluid chemistry Melted surface samples and supraglacial stream water samples were
                    filtered using 0.22 μm single use syringe filters into acid-washed Nalgene
                    bottles. Inductively-coupled plasma mass spectroscopy (ICP-MS; Thermo Fisher
                    iCAPQc) was used to measure fluid phase cations in the filtered water samples
                    that were acidified using Aristar HNO 3 . ICP-MS was
                    conducted by Stephen Reid at the University of Leeds, UK. Phosphorus was either
                    measured using segmented flow-injection analysis (AutoAnalyser3, Seal
                    Analytical), or for samples containing lower concentration of phosphorus using a
                    100 cm WPI Liquid Waveguide Capillary Cell in conjunction with an Ocean Optics
                    USB2000 + spectrophotometer with a precision of 1.6% and a LOD of
                        2 nmol L −1 . Aliquots of the non-acidified 0.22 μm
                    filtered samples were also analyzed in replicates by ion chromatography by
                    Andrea Viet-Hillebrand at the German Research Centre for Geosciences, Potsdam,
                    Germany. Analyses were carried out with a conductivity detector on a Dionex ICS
                    3000 system, equipped with an AS 11 HC Dionex analytical column run at 35 °C for
                    chromatographic separation of the anions. Standards containing all investigated
                    inorganic ions (F − , Cl − ,
                        SO 4 2− ,
                        NO 3 − ,
                        PO 4 3− ) were analyzed and
                    all replicate samples had a standard deviation <10%. Detailed results
                    can be found in Supplementary Table 8 . Carbon and nitrogen content Aliquots from the 0.7 µm GFF filtered, dried and hand-milled
                    samples were analyzed for their bulk total and organic carbon (TC and TOC) and
                    total nitrogen (TN) content. This was done for the H bio ice, DCC ice, H bio snow, and cryoconite hole material
                    using an elemental analyzer (NC2500 Carlo Erba, standard deviation < 0.2
                    %, precision 0.1 %) and with the TOC concentrations subsequently measured
                    following an in situ decalcification step. Note, the organic carbon fraction
                    includes a contribution from black carbon. TC/TN analyses were conducted by
                    Birgit Plessen and Sylvia Pinkerneil at the German Research Centre for
                    Geosciences, Potsdam, Germany. Detailed results found in Supplementary
                        Table 5 . Pearson’s product-moment
                    correlation r -values in Fig. 3 and supplementary Fig. 2 were calculated using Excel (v16.xx). Mineralogy The mineralogy of the dust was determined using a Bruker D8 Advance
                    Eco X-ray diffractometer (Bruker, Billerica, USA) with a Cu source, operated at
                    40 kV and 40 mA at the University of Leeds, UK. Samples were hand-milled in an
                    agate mortar and pestle prior to loading in 5 or 10 mm low-background silicon
                    mounts. The small quantity of material per sample necessitated the use of
                    shallow sample mounts, thereby making the sample not infinitely thick with
                    respect to X-rays, and thus rendering this analysis semi-quantitative. Furthermore, because it was necessary to rely on hand grinding, XRD patterns
                    exhibit the effects of non-ideal particle size statistics and preferred
                    orientation on some phases, which can result in higher
                        R wp values. The 2016 COD and 1996 ICDD databases were
                    used to complete phase identification for each sample, in conjunction with
                            DIFFRAC plus Eva v.2 software [56] . Topas V
                            4.2 [56] and the fundamental parameters
                            approach [57] were used to complete Rietveld
                            refinements [25] , [58] , [59] . No preferred orientation corrections were
                    used because refinements are typically more accurate for samples containing many
                    phases that are known to exhibit severe preferred orientation (e.g.,
                    phyllosilicates) when such corrections are excluded [60] . In some cases, the use
                    of multiple K-feldspar, plagioclase feldspar, and orthopyroxene structures were
                    used in a single refinement because this approach provided substantially
                    improved fit statistics and visual fits to observed XRD patterns. This may
                    reflect the incorporation of dust from multiple source rocks of differing
                    mineralogical composition. Mineral phases identified using XRD were grouped into
                    the following classes: quartz, plagioclase feldspars
                    (albite/andesine/anorthite), amphiboles (refined using the structure of
                    actinolite), potassium feldspars (orthoclase/microcline), pyroxene
                    (enstatite/augite/diopside), and micas (refined using the structure of
                    muscovite). Detailed results are found in Supplementary Tables 6 and 7 . Microbial community composition A total of 26 samples comprising 15 high algal biomass ice
                        (H bio ice), two high algal biomass snow (Hbio_snow),
                    one biofilm, four dispersed cryoconite (DCC) (macroscopically visible
                    particles), and four clean ice (CI) samples (without macroscopically visible
                    particles) were collected into sterile 50 mL centrifuge tubes
                        (H bio ice, H bio snow, DCC,
                    Biofilm) or sterile sampling bags (CI). After gentle thawing at field-lab
                    temperatures (~5–10 °C), and concentrating by gravimetric settling of particles
                    (for H bio ice, H bio snow, DCC,
                    Biofilm) or filtering (CI) through sterile Nalgene single-use filtration units
                    (pore size 0.22 µm), up to 5 replicate from the concentrates or 1 filter per
                    sampling event were transferred to 5 ml cryo-tubes and immediately frozen in
                    liquid nitrogen. Samples were returned to the German Research Centre for
                    Geosciences in Potsdam, Germany in a cryo-shipper at liquid nitrogen
                    temperatures and stored at −80 °C until processing. DNA was extracted from all samples using the PowerSoil
                        (H bio ice, H bio snow, DCC,
                    Biofilm) or PowerWater (CI) DNA Isolation kits (MoBio Laboratories). The 16 S
                    rRNA, 18 S rRNA and ITS amplicons were prepared according to the Illumina “16 S
                    Metagenomic Sequencing Library Preparation” guide. 16 S rRNA genes were
                    amplified using the bacterial primers 341 F (5′-CCTACGGGNGGCWGCAG) and 785 R
                    (5′-GACTACHVGGGTATCTAATCC) spanning the V3-V4 hypervariable regions. 18 S rRNA
                    genes were amplified using the eukaryotic primers 528 F (5′ GCGGTAATTCCAGCTCCAA)
                    and 706 R (5’ AATCCRAGAATTTCACCTCT; Cheung et al., 2010) spanning the V4-V5
                    hypervariable regions. ITS amplicons were amplified using the primers 5.8SbF (5′
                    CGATGAAGAACGCAGCG) and ITS4R (5′ TCCTCCGCTTATTGATATGC) spanning the ITS2 region. All primers were tagged with the Illumina adapter sequences. Polymerase chain
                    reactions (PCR) were performed using KAPA HiFi HotStart ReadyMix. Initial
                    denaturation at 95 °C for 3 min was followed by 25 cycles of denaturation at
                    95 °C for 30 s, annealing at 55 °C for 30 s, and elongation at 72 °C for 30 s.
                    The final elongation was at 72 °C for 5 min. All PCRs were carried out in
                    reaction volumes of 25 µL. All pre-amplification steps were done in a laminar
                    flow hood with DNA-free certified plastic ware and filter tips. Amplicons were
                    barcoded using the Nextera XT Index kit. The pooled library was sequenced on the
                    Illumina MiSeq using paired 300-bp reads at the University of Bristol Genomics
                    Facility, Bristol, UK. The sequenced 16 S, 18 S, and ITS2 libraries were individually
                    imported into Qiime2 (v.2019.1) [61] . Itsxpress was used to extract the
                    precise ITS2 region, and thus removing the conserved regions, from the ITS2
                    libraries before further processing (--p-region ITS2, _--p-taxa ALL). The
                    imported libraries were quality-filtered using the dada2 pipeline (16 S:
                    --p-trunc-len-f = 280, --p-trunc-len-r = 200, --p-trim-feft-f = 10,
                    --p-trim-left-r = 10; 18 S: --p-trunc-len-f = 250, --p-trunc-len-r = 200,
                    --p-trim-feft-f = 10, --p-trim-left-r = 10; ITS2: --p-trunc-len-f = 0,
                    --p-trunc-len-r = 0, --p-trim-feft-f = 0, --p-trim-left-r = 0). The amplicon
                    sequence variants (ASV) in the filtered libraries were classified using
                    classify-sklearn and the respective databases Greengenes (16 S,
                            “gg-13-8-99-nb-classifier”) [62] , Silva (18 S,
                            “silva-132-99-nb-classifier”) [63] , and Unite (ITS2,
                            “unite_ver8_99_02.02.2019”) [64] . ASVs skewing the results were removed
                    from each data set (16 S: --p-exclude Chloroplast, mitochondria; 18 S:
                    --p-exclude Archaea, Bacteria). Feature tables containing solely algal (18 S:
                    --p-include Chloroplastida, Ochrophyta) or fungal (ITS2: --p-include Fungi)
                    sequences were created. Subsequently, all feature tables were rarefied to the
                    lowest yet sufficient sample size and low-coverage samples below this threshold
                    were discarded (16 S: 5500, ITS2: 15000, 18 S: 15000). Further, only ASVs with a
                    minimum frequency count of 10 were retained in the feature tables. Detailed
                    results can be found in Supplementary Tables 9 – 13 . The filtered feature tables were imported into R (v.3.6.0) to
                    create bar charts representing the respective community compositions based on
                    their relative abundances. Non-metric multidimensional scaling (NMDS) analyses
                    were performed using the “metaMDS” function (Bray-Curtis distances) of the R
                    package “vegan” and plots were created using the package “ggplot2”. Analysis of
                    similarities (ANOSIM) was carried out using the “anosim” function of the “vegan”
                    package and “sites” and “habitats” as treatment groups. Scanning electron microscopy (SEM) H bio ice, cryoconite, DCC ice, and biofilm
                    samples were fixed using 2.5 % v/v glutaraldehyde and stored at 4 °C. Samples
                    were dehydrated via an ethanol dehydration series (25%, 50%, 75%, 100%, 100%,
                    100%) for 15 min at each step, followed by 10 min in each of: 50:50 ethanol:
                    hexamethyldisilazane (HMDS), and 2 × 100% HMDS. The HMDS was removed and the
                    samples were air-dried prior to being mounted on stainless steel stubs using
                    adhesive carbon tabs. Samples were coated with 5 nm of iridium using an Agar
                    High Resolution sputter coater. SEM characterization of the samples was
                    conducted using a Hitatchi 8230 SEM at the Leeds Electron Microscopy and
                    Spectroscopy Centre (LEMAS), University of Leeds, UK. Rare Earth Element analysis and data compilation Rare Earth Element (REE) analysis was conducted on
                        H bio ice, DCC ice, and cryoconite hole particulate
                    solid materials filtered onto 0.7 µm GFF and hand-milled in an agate mortar and
                    pestle. To remove organic matter, samples were ashed in a slightly open ceramic
                    crucible in a muffle furnace at 450 °C for 4 h. Rock samples collected from site
                    6 by Gilda Varliero and Gary Barker (University of Bristol, UK) (representing
                    lithologies of the catchment area) were cut into centimeter-sized cubes prior to
                    milling in a tungsten ring mill. Acid dissolution of the mineral fraction was
                    achieved in Savillex® beakers using pro-analysis acids previously purified by
                    distillation and sub-boiling. Dissolution was first performed with 2 mL 14 M
                        HNO 3 and 1 mL 23 M HF on a hot plate at 120 °C for
                    48 h and later, after evaporation to dryness, with 2 mL 6 M HCl on a hot plate
                    at 120 °C for 24 h. REE concentrations were determined using HR-ICP-MS
                    (ThermoFisher Element 2) at the Vrije Universiteit Brussel, Belgium. Trace
                    element concentrations were calibrated using elemental standard solutions and
                    USGS reference material (AGV-2). Precision for all elements is better than 2%
                    RSD. Detailed results can be found in Supplementary Table 14 . Mineral dust particle size distribution analysis Approximately 100 mg of each sample was transferred to a 50 mL
                    centrifuge tube, to which 35 mL of 30%
                        H 2 O 2 (w/w) (Honeywell Fluka™)
                    was added in order to remove the organic content. The tubes were sonicated (VWR
                    ultrasonic cleaner) for 10 min to disaggregate the solids. The samples were
                    agitated in an orbital shaking incubator operating at 100 rpm at 35 °C. After
                    72 h, the samples were centrifuged at 4000 rpm for 10 min (Eppendorf centrifuge
                    5810). The supernatant was removed and replaced with new
                        H 2 O 2 . This was repeated six
                    times until no more organic oxidation was observed. The mineral fraction was
                    washed three times in water (Sartorius arium pro ultrapure water) for 24 h, with
                    centrifugation succeeding each wash. The organic-free mineral fractions were
                    dried at 35 °C prior to particle size analysis measured by Kerstin Jurkschat
                    using a DC24000 CPS disc centrifuge [65] at Oxford Materials Characterisation
                    Services, Oxford, UK. LAP mass loading quantification Aliquots of melted snow and ice samples of known volumes were
                    filtered in the field successively through pre-weighed 5 μm and 0.2 μm
                    polycarbonate filters. The filters were returned to the University of Leeds, UK
                    where they were dried and weighed to determine the mass of LAP per volume of
                    melted sample. The sum of the total organic carbon and nitrogen was used as a
                    proxy to indicate the biomass fraction of each sample, with the remaining sample
                    mass allocated to mineral dust. These values were used to calculate the mineral
                    dust mass loading per unit of melted ice. Reporting summary Further information on research design is available in
                        the Nature Research Reporting
                        Summary linked to this article.